Waveguide integrated superconducting single-photon detectors implemented as near-perfect absorbers of coherent radiation At the core of an ideal single-photon detector is an active material that absorbs and converts every incident photon to a discriminable signal. A large active material favours efficient absorption, but often at the expense of conversion efficiency, noise, speed and timing accuracy. In this work, short (8.5 μm long) and narrow (8 × 35 nm 2 ) U-shaped NbTiN nanowires atop silicon-on-insulator waveguides are embedded in asymmetric nanobeam cavities that render them as near-perfect absorbers despite their small volume. At 2.05 K, when biased at 0.9 of the critical current, the resulting superconducting single-photon detectors achieve a near-unity on-chip quantum efficiency for ∼ 1,545 nm photons, an intrinsic dark count rate <0.1 Hz, a reset time of ∼ 7 ns, and a timing jitter of ∼ 55 ps full-width at half-maximum. Such ultracompact, high-performance detectors are essential for progress in integrated quantum optics. Over the past decade, photonic quantum information processing [1] , [2] has shown considerable promise for quantum computing [3] , [4] , [5] , communication [6] and metrology [7] , [8] , [9] . Most of the impressive proof-of-principle demonstrations have relied on bulk optics [2] that is inherently non scalable [10] . Independent progress on conventional integrated photonic circuitry [11] , [12] , [13] , [14] suggests that integrated quantum photonic circuits [10] may offer a scalable solution. A variety of pertinent host material systems [15] , [16] , [17] , [18] , [19] , [20] , [21] are being studied, but the unparalleled recent progress in classical silicon-based photonic circuits [12] , [22] , [23] , [24] makes silicon particularly attractive. Phase modulators and a wide assortment of ultracompact (tunable) passive components have been demonstrated in the silicon-on-insulator (SOI) platform [25] . Already some of these have been integrated [26] , [27] with on-chip entangled and heralded photon sources [28] , [29] , [30] , [31] , [32] , [33] , [34] , single-photon detectors [35] , and used to demonstrate quantum interference and manipulation [36] , [37] . All the optical components on a SOI platform—including the detectors—should operate at telecommunications compatible infrared wavelengths. Superconducting nanowire single-photon detectors (SNSPD) [38] , [39] represent the most promising stand-alone infrared photon counting technology, and so it is not surprising that nanowires placed on top of optical waveguides have figured prominently in recent demonstrations of integrated single-photon detectors [35] , [40] , [41] , [42] , [43] , [44] . In the travelling wave (TW) configuration employed in these detectors, photons propagating down micron-wide waveguides are evanescently absorbed by a critically biased superconducting nanowire over a distance of tens of microns, and then an easily detectable normal-state transition in the nanowire occurs [39] . Various of TW SNSPDs have achieved high quantum efficiencies (up to 91% ref. 35 ), or low noise (down to <0.01 Hz [45] ), or fast recovery time (<10 ns [35] ), or accurate timing response (<20 ps of jitter [35] ), but no single integrated detector in a fixed operation condition performs well in all of these critical categories. If truly scalable quantum information on-a-chip is to become practical, then detectors that excel in all of these individual performance metrics are needed. The evanescent absorption in the TW geometry intrinsically puts a minimum on the coupling length of an efficient detector, and correspondingly, the length of the nanowire (typically between 40 and 400 μm [35] , [41] , [42] depending on the nanowire layout and the host material system). A higher packing density of lower noise [46] , faster [47] , [48] and more accurate detectors [49] should be possible if the nanowire length could be further reduced. The obvious challenge is the apparent trade-off with absorption efficiency [50] (shorter wires offer less absorbing volume). This paper describes a successful strategy for circumventing this trade-off, by embedding a short (8.5 μm) ultranarrow (8 × 35 nm 2 ) superconducting nanowire within a high-quality factor microcavity specifically designed to turn the overall detector into a near-perfect absorber of coherent radiation [51] , [52] , [53] . Implemented on a SOI platform, the detector’s ultrasmall footprint (0.5 × 7.0 μm 2 )—smaller than any reported to date—also incorporates a built-in optical filter. It absorbs and detects nearly all of the ∼ 1,545 nm light in the waveguide, exhibits a sub-Hz intrinsic dark count rate, has a fast recovery time of ∼ 7 ns, and shows a small timing jitter of ∼ 55 ps full-width at half-maximum (FWHM). The latter timing quantities are consistent with limitations imposed by the readout electronics, which have not been optimized. This ultracompact integrated detector therefore achieves a comprehensive set of metrics that are all either close to ideal or comparable to the best of class that have been reported using various implementations of infrared single-photon detectors. Design concept In order for a short nanowire to absorb virtually every photon incident along a waveguide, it is placed within an asymmetric optical microcavity defined by etching a series of holes on either side of the nanowire (see scanning electron microscope images (SEM) in Fig. 1a,b ). The cavity containing the weakly absorbing nanowire is designed to function as a coherent perfect absorber [51] , [52] , [53] . Figure 2a shows a model of the cavity. 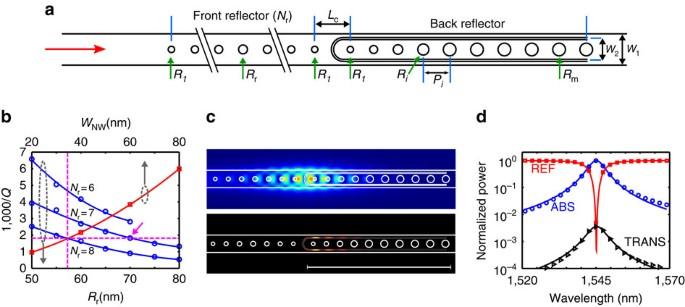Figure 2: Design of an integrated microcavity SNSPD. (a) Model for an asymmetric nanobeam cavity enclosing a nanowire. Fixed parameters are: silicon waveguide width (W1=500 nm); nanowire layout (W2=350 nm); design of the back reflector (maximum hole radiusRm=100 nm); minimum hole radius (R1=50 nm); and cavity length (Lc=560 nm). Variable parameters are: number of holes (Nr) and maximum hole radius (Rr) of the front reflector, and nanowire widthWNW. For the pitch,Pi=1.22Ri+308 nm is used to center the photonic bandgap to 1,545 nm. The tapers are linear. (b) SimulatedQA(WNW) (red squares), andQr(Rr,Nr) (blue circles). The solid lines are the best polynomial fits. The dashed lines and pink arrow mark the design of microcavity SNSPDs presented in this paper. (c) Simulated magnitude of the electric field on the waveguide surface (top) and power dissipation density in the nanowire (bottom) for a microcavity SNSPD (WNW=35 nm,Nr=7,Rr=70 nm) excited with TE-polarized 1,545 nm guided light from the left. Scale bar, 4 μm. (d) Simulated absorption (ABS—blue circles), reflection (REF—red squares) and transmission (TRANS—black triangles) for the same device. The lines are Lorentzian fits. Ideally (ignoring all other losses), the reflectivity of the back mirror (right side) is unity, so all of the light incident from the left must be either absorbed or reflected. At the resonant frequency of the cavity, ω R , a portion of the light incident from the left excites a resonating cavity mode with amplitude A . The normalized power reflected back into the incident waveguide is then , and the power absorbed by the nanowire is 2| A | 2 / τ A , where τ r and τ A are the time constants associated with the decay of A into the waveguide and the nanowire, respectively [54] . Power conservation in this idealized scenario requires , which in general determines how much of the incident light reflects, and how much is transferred into the cavity. 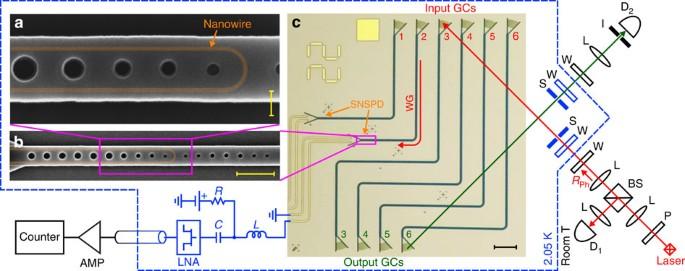However, if the left side mirror reflectivity is designed such that τ r = τ A , then all of the incident light is perfectly transferred to the cavity and absorbed. Figure 1: A waveguide integrated SNSPD designed as a near-perfect absorber of coherent radiation. (a) Enlarged scanning electron microscope image of the detector (nanowire is coloured) showing the nanowire geometry and the photonic crystal holes. Scale bar, 200 nm. (b) Zoomed out image showing the entire nanowire and the cavity. Scale bar, 1 μm. (c) Optical micrograph of a typical chip that includes two SNSPDs connected to grating couplers (GC) number 1 and 2 via two waveguides (WG). Scale bar, 50 μm. The other devices are for calibration purposes. The rest of the figure shows the characterization setup. The dashed blue line encloses components held at cryogenic temperature (2.05 K). The photons generated by a laser are delivered to the detector through waveguides, grating couplers, a hole in a cold shield surrounding the chip (S) and room-temperature optics (P, polarizer; L, lens; BS, beam-splitter; W, cryostat windows; D1, power meter). GC–WG–GC devices together with a second set of room temperature optics that involves D2are used for calibration, imaging and alignment purposes (I, iris). The nanowire is biased by a voltage source, a resistor (R=100 Ω), and an inductor (L=100 nH). The detection signal is delivered to a low noise amplifier (LNA) through a coupling capacitor (C=22 pF) for transmission to a room temperature amplifier (AMP) and a counter through a coaxial cable. Figure 1: A waveguide integrated SNSPD designed as a near-perfect absorber of coherent radiation. ( a ) Enlarged scanning electron microscope image of the detector (nanowire is coloured) showing the nanowire geometry and the photonic crystal holes. Scale bar, 200 nm. ( b ) Zoomed out image showing the entire nanowire and the cavity. Scale bar, 1 μm. ( c ) Optical micrograph of a typical chip that includes two SNSPDs connected to grating couplers (GC) number 1 and 2 via two waveguides (WG). Scale bar, 50 μm. The other devices are for calibration purposes. The rest of the figure shows the characterization setup. The dashed blue line encloses components held at cryogenic temperature (2.05 K). The photons generated by a laser are delivered to the detector through waveguides, grating couplers, a hole in a cold shield surrounding the chip (S) and room-temperature optics (P, polarizer; L, lens; BS, beam-splitter; W, cryostat windows; D 1 , power meter). GC–WG–GC devices together with a second set of room temperature optics that involves D 2 are used for calibration, imaging and alignment purposes (I, iris). The nanowire is biased by a voltage source, a resistor ( R =100 Ω), and an inductor ( L =100 nH). The detection signal is delivered to a low noise amplifier (LNA) through a coupling capacitor ( C =22 pF) for transmission to a room temperature amplifier (AMP) and a counter through a coaxial cable. Full size image Figure 2: Design of an integrated microcavity SNSPD. ( a ) Model for an asymmetric nanobeam cavity enclosing a nanowire. Fixed parameters are: silicon waveguide width ( W 1 =500 nm); nanowire layout ( W 2 =350 nm); design of the back reflector (maximum hole radius R m =100 nm); minimum hole radius ( R 1 =50 nm); and cavity length ( L c =560 nm). Variable parameters are: number of holes ( N r ) and maximum hole radius ( R r ) of the front reflector, and nanowire width W NW . For the pitch, P i =1.22 R i +308 nm is used to center the photonic bandgap to 1,545 nm. The tapers are linear. ( b ) Simulated Q A ( W NW ) (red squares), and Q r ( R r , N r ) (blue circles). The solid lines are the best polynomial fits. The dashed lines and pink arrow mark the design of microcavity SNSPDs presented in this paper. ( c ) Simulated magnitude of the electric field on the waveguide surface (top) and power dissipation density in the nanowire (bottom) for a microcavity SNSPD ( W NW =35 nm, N r =7, R r =70 nm) excited with TE-polarized 1,545 nm guided light from the left. Scale bar, 4 μm. ( d ) Simulated absorption (ABS—blue circles), reflection (REF—red squares) and transmission (TRANS—black triangles) for the same device. The lines are Lorentzian fits. Full size image In the ideal scenario above, an arbitrarily short nanowire (arbitrarily long τ A ) can absorb all of the incident radiation as long as the reflectivity of the input mirror can be precisely tuned close to 100% (that is, a very long τ r ). In practice, there will also be some additional scattering losses associated with the cavity, so its overall quality factor, Q will be given by , where Q A = ω R τ A /2, and Q r = ω R τ r /2. The above analysis indicates that detectors with absorption efficiency η A ∼ 1, can be achieved using very short and narrow nanowires as long as dielectric reflectors can be designed such that Q A = Q r << Q scatt . The minimum nanowire length ( L NW ) is dictated by how tightly localized the high Q scatt cavity mode is, and therefore high-index contrast host materials like SOI are ideal. Finally, it is noted that this approach necessarily limits the bandwidth over which the detector absorbs efficiently, to ∼ ω R / Q . However, for many quantum information processing applications, optical filters are placed in front of detectors to minimize spurious counts due to stray photons [55] , [56] . The near-perfect absorber detector design described here actually integrates the filter and detector into a single, compact unit. Design details The microcavity SNSPDs are formed by patterning holes in a silicon nanobeam (silicon on SiO 2 , 190-nm thick, 500-nm wide) to form an asymmetric cavity around a U-shaped nanowire (NbTiN, 8 nm thick, W NW wide) that lies on top of the nanobeam, as illustrated in Fig. 2a . Nanobeam cavities [54] , [57] allow low-loss coupling to waveguides, high Q scatt , low mode volume and an accessible near field that are all useful features for microcavity SNSPDs. The back (perfect) reflector consists of 10 holes, 6 of fixed radius ( R m =100 nm) and 4 with shrinking radii, down to R 1 =50 nm, towards the input waveguide to impedance match the Bloch mode to the waveguide mode. The front (partial) reflector has N r holes, all of which are linearly tapered from a maximum hole radius of R r down to R 1 =50 nm on both sides. These one-dimensional photonic crystals [54] were designed (see simulation Methods) to have a bandgap centered at 1,545 nm. To design the microcavity, N r =14 and R r =100 nm are fixed, and the cavity length ( L c ) in the absence of the nanowire is adjusted to get a mode at the detector operation wavelength of 1,545 nm with a moderate Q =5.6 × 10 4 . This ensures appropriate design of tapers and consequently a high enough Q scatt >5.6 × 10 4 . When the nanowire is added to the same cavity, the mode profile and wavelength stay almost fixed, but the new Q ≃ Q A ( W NW ) is substantially reduced, even for the smallest W NW =20 nm (see squares in Fig. 2b ). Removing the nanowire and reducing R r and N r results in a new set of Q ≃ Q r ( R r , N r ), with values comparable to Q A ( W NW ) (see circles on Fig. 2b ). A nanowire with a certain W NW (for example, vertical dashed line in Fig. 2b ) and thus fixed Q A (horizontal dashed line) will absorb almost all incident coherent light if N r and R r are chosen such that Q r ( R r , N r )= Q A ( W NW ) (pink arrow in the same figure). Note that in this design algorithm, L NW is fixed by what is required for electrical connection through the back reflector ( ∼ 2 × 4 μm); this can in principle be further reduced by employing a better connection topology. The fabricated microcavity SNSPDs have nominal parameters; W NW =35 nm, N r =7, R r =70 nm, , and L NW =8.5 μm. The distributions of electric field and power loss are as shown in Fig. 2c , for the structure excited with the mode of the strip waveguide at 1,545 nm. The field is tightly localized by the cavity, and the absorption is concentrated over a micron-length portion of the nanowire. At resonance, the calculated absorption peaks at 98.4%, while reflection, transmission and radiated losses are 0.04, 0.3 and 1.1%, respectively (see simulated spectrum shown in Fig. 2d ). Analysing the variation of peak absorption with different fabrication imperfections ( Supplementary Note 1 , Supplementary Table 1 ) shows the structure is quite robust. Analysis of the radiation losses shows that 1% of the total 1.1% is lost to the substrate. Q scatt could therefore be further increased by undercutting the nanobeam, and the back-transmission could be further reduced by adding more holes. Applying both strategies, the losses would be reduced to ∼ 0.2% and the absorption could peak close to ∼ 99.8%. For comparison, the simulated absorption of the same 8.5 μm long nanowire, but without the cavity, is 29%; a 160 μm long nanowire would be needed to obtain 99.8% absorption in the absence of the cavity. The huge reduction of L NW without compromising absorption efficiency ( η A ) promises fewer dark counts, and a more compact footprint for an efficient high-speed detector, as demonstrated and discussed below. Measurement set-up Figure 1c is a micrograph showing a portion of one of the fabricated chips. It consists of detectors with input waveguides connected to focusing grating couplers [58] (GC) as well as gold electrical connections that are routed to large contact pads (not shown). Also included on the chip are devices with two GCs connected by a waveguide; these were used for alignment and calibration purposes. The chip was installed on, and wire-bonded to, a custom-made printed circuit board that hosts electronic circuits to apply bias, preamplify the detection signal and impedance match the detector to a 50 Ω coaxial cable that runs to room-temperature amplifiers and then to a counter (see schematics in Fig. 1 ). The board was installed in an optical cryostat (SVT-300, Janis Inc.) where it was submerged in superfluid helium ( T =2.05 K). The whole-sample holder is surrounded by a cylindrical brass shield with two holes (S in Fig. 1 ) of 6 mm diameter coaxial with the two 45° windows (W in Fig. 1 ), one for the excitation laser light, and the other to image the chip for aligning and calibration. An attenuated and polarization-controlled continuous-wave tunable laser (TLB-6600, New Focus Inc.) was coupled to waveguides by focusing it on the input grating couplers. The setup was calibrated to read the rate of photons incident through the input cryostat window ( R Ph in Fig. 1 ) by the power meter D 1 (see Supplementary Note 2 and Supplementary Fig. 1 for details). Efficiency and dark count characterization To measure the quantum efficiency and noise performance, three different count rates were determined (see Methods): photon count rate (PCR) measured when the input grating couplers were excited by the laser; background (mostly blackbody) count rate (BCR, also called system dark count rate) measured in the same conditions but with the laser off; and dark count rate (DCR, also called intrinsic dark count rate) measured when a cylindrical brass shield (50 μm thick) without any holes surrounded the sample holder. The BCR will exceed the DCR because the large cryostat windows—which were unshielded for PCR and BCR measurements—allow intense black body radiation to enter the cryostat. The quantum efficiency (QE= η A η D , where η D is the bias-dependent efficiency of converting absorbed photons to electric pulses) was deduced from the measured rates as (PCR−BCR)/( η C R Ph ), where η C is the efficiency of coupling the incident photons ( R Ph ) into the strip waveguides. 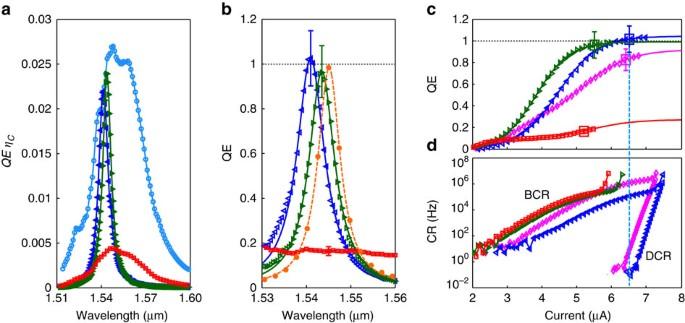Figure 3: Integrated SNSPD detection performance. Each symbol represents a fixed device throughout the figure. (a)QEηCmeasured over a wide bandwidth for detectors biased at∼0.9IC. Triangles are for microcavity SNSPDs; squares are for a TW-based detector withLNW=8.5 μm (that is, the same nanowire of microcavity detectors but without cavity holes); circles are forηC(that is,QE=1). (b) On-chip QE versus wavelength at∼0.9IC. The solid lines drawn on triangles are the best Lorentzian fits to measured data. Filled-circles are the simulatedηA; and a dashed line on filled-circles shows the best Lorentzian fit to simulated data. Dotted line at 1.0 is merely for guiding the eye. (c) QE versus bias current measured at the cavity resonance wavelength for microcavity SNPSDs (triangles), and at 1,550 nm for TW SNSPDs (squares forLNW=8.5 μm, diamonds forLNW=57.2 μm). For each device,∼0.9ICis marked by a square. The solid lines are the best sigmoidal fits. (d) DCR and BCR measured versus bias current. The vertical dashed line marks∼0.9ICfor a microcavity SNSPD and is merely for guiding the eye. All the detector measurements were done at 2.05 K. The error bars show one s.d. uncertainty equal to ±8%. Figure 3a shows the system quantum efficiency, QE η C , for several SNSPDs, all biased at a current equal to ∼ 0.9 of the experimentally determined critical current ( I C ). Triangles are for two microcavity SNSPDs, while squares are for a device with the same nanowire layout, but without any cavity holes, effectively a TW structure. In contrast with the TW device that exhibits a broad spectral response, the microcavity devices show a resonant response. Note that the off-resonant QE η C goes to negligibly small values compared with the peak (only 0.3% of the peak QE η C ), confirming negligible contribution of non-guided photons to the peak PCR. Figure 3: Integrated SNSPD detection performance. Each symbol represents a fixed device throughout the figure. ( a ) QEη C measured over a wide bandwidth for detectors biased at ∼ 0.9 I C . Triangles are for microcavity SNSPDs; squares are for a TW-based detector with L NW =8.5 μm (that is, the same nanowire of microcavity detectors but without cavity holes); circles are for η C (that is, QE =1). ( b ) On-chip QE versus wavelength at ∼ 0.9 I C . The solid lines drawn on triangles are the best Lorentzian fits to measured data. Filled-circles are the simulated η A ; and a dashed line on filled-circles shows the best Lorentzian fit to simulated data. Dotted line at 1.0 is merely for guiding the eye. ( c ) QE versus bias current measured at the cavity resonance wavelength for microcavity SNPSDs (triangles), and at 1,550 nm for TW SNSPDs (squares for L NW =8.5 μm, diamonds for L NW =57.2 μm). For each device, ∼ 0.9 I C is marked by a square. The solid lines are the best sigmoidal fits. ( d ) DCR and BCR measured versus bias current. The vertical dashed line marks ∼ 0.9 I C for a microcavity SNSPD and is merely for guiding the eye. All the detector measurements were done at 2.05 K. The error bars show one s.d. uncertainty equal to ±8%. Full size image The overall system efficiency numbers reported in Fig. 3a are small mainly due to the low grating coupling efficiency, and waveguide propagation losses. A far more relevant metric for integrated quantum optics applications is QE, the efficiency of detecting waveguided photons that are incident on the partial reflector of the microcavity SNSPDs (or the bare nanowire in the case of the TW devices). Therefore, a measurement of η C is needed to normalize the QEη C values reported in Fig. 3a to get the QE. As discussed in Methods: (i) η C ( λ ) is determined up to a scaling constant, (asymptotic saturated value of η D at high bias currents), by normalizing to the single-photon count rate from a reference TW SNSPD, (ii) η C ( λ ) is fully determined using a detailed analysis of all the losses experienced by photons focused into the cryostat, before reaching the integrated SNSPDs. The final results are: (i) η C ( λ ) shown by circles in Fig. 3a (the one s.d. uncertainty is ±8%); and (ii) for the reference TW SNSPD studied in this analysis, to one s.d. of uncertainty. The on-chip QEs at ∼ 0.9 I C shown in Fig. 3b (with the same symbol conventions of Fig. 3a ) were thus obtained by dividing the respective curves in Fig. 3a by η C . The QEs for the two microcavity SNSPDs peak close to unity (1.02±8% and 0.97±8%). The nominal peak QE for one of the microcavity devices exceeds unity, but values as low as 1.02−0.08=0.94 are also consistent with the one sigma statistical uncertainty associated with the measurements. The peak QEs for the microcavity devices at ∼ 0.9 I C are consistent with η A close to unity, as expected from simulations and further discussed below. Note that the QE for the device without the cavity stays flat and small, consistent with the broadband nature of both η A and η D [59] , and the relatively low η A for this particular TW device that consists of a relatively short nanowire. Shown on the same figure, with filled circles and a dashed line (best Lorentzian fit), is the simulated η A for the designed microcavity detector. The spectral line shapes of the fabricated microcavity devices are close to the designed line shape, but blue shifted (the resonant wavelengths are 1,541 nm and 1,543 nm compared with target value of 1,545 nm.). This slight discrepancy is most likely due to the uncertainty associated with the physical dimensions of the waveguide used in the simulations, given the high sensitivity of the resonant wavelength on the geometry (for example, a 1 nm change in waveguide width results in a ∼ 1 nm shift in resonant frequency, as shown in the Supplementary Table 1 ). In addition to wavelength, the quantum efficiency of a microcavity SNSPD is a function of bias current. Figure 3c shows the QE versus bias current at a fixed wavelength for the same devices with the same symbols. The bias current of ∼ 0.9 I C used for each device reported in Fig. 3a,b is marked with a large square. The QEs of the two microcavity devices (triangles) measured at the resonant frequencies follow a single sigmoidal line shape (see solid red lines on the triangles). These QEs at ∼ 0.9 I C are both ∼ 2% smaller than their respective saturation levels at 1.04 and 0.99. This suggests an η D at ∼ 0.9 I C as high as . As noted above, the calculated peak η A is at most 0.984, so even for a microcavity SNSPD with an ideal , the highest possible QE at 0.9 I C will be QE = η A η D < ∼ 0.984 × 0.98= ∼ 0.96. This is consistently within the one s.d. uncertainty of the nominal values of the measured QEs. The QE for an 8.5 μm long nanowire device without a cavity (squares on Fig. 3c ) measured at 1,550 nm follows a more complex dependence on bias current, signalling the presence of a material or geometrical constriction in the nanowire (consistent with its smaller I C ). Investigating the nanowires of this work under an SEM revealed the presence of an asymmetry in some of the fabricated nanowires: the two parallel branches that make a U-shape have slightly (approximately few nanometer) different widths. Therefore, a double sigmoidal curve (one sigmoid for each branch) possibly explains the response of such devices. The result of this fit is shown by a solid red line on the squares of Fig. 3c . The fitted sigmoid has a saturation at QE=0.27, close to the simulated η A of 0.29. The electron-beam lithography step was identified as the cause of this width asymmetry, and reducing the pattern writing speed helped mitigate the effect. However, more experimental tuning is still needed to completely resolve the problem. For comparison, a TW device with a simulated η A of 0.90 was also fabricated using a relatively long nanowire ( W NW =35 nm) length of 57.2 μm. The QE of this device (diamonds in Fig. 3c ) changes considerably more gradually with the bias current than the microcavity structures; such that at ∼ 0.9 I C the QE is 0.89 of its saturated level at ∼ 0.92. Therefore, compared with the microcavity devices with , the QE of this long nanowire device is reduced both because of the smaller η A , and the relatively poor saturation behaviour of the η D ( I B ). The above relatively poor performance of the longer nanowire in the TW geometry most probably reflects the inevitable non-uniformities (both in geometry and superconducting material properties) along the nanowire. This can cause non-uniformity in the η D ( I B ) values for photons absorbed by different sections of a nanowire carrying a fixed bias current of I B . The difference of the two detector structures is that in a microcavity device optical absorption is highly focused on a very short nanowire length (see power dissipation density plot of Fig. 2c ), and therefore the QE( I B ) depends on the η D ( I B ) of a very short length of the nanowire. In contrast, the optical absorption in a TW device takes place over a much longer nanowire length, and therefore the QE( I B ) is smoothed by averaging the η D ( I B ) values over a longer length. The present hypothesis suggests another possible advantage of reducing L NW in microcavity detectors: it helps achieve high η D in addition to high η A , and therefore a high QE. Quite apart from being efficient, a good detector must exhibit low noise. Figure 3d shows DCR and BCR measurements for the devices of Fig. 3c with the same symbols. The DCR starts from a plateau-like level at around 0.1 Hz followed by a fast exponential increase as expected for nanowire detectors. The plateau likely originates from black-body radiation that enters the cryostat from the top or even through the thin brass foil; it could be reduced by using better shields [45] , [55] . At ∼ 0.9 I C the DCR for the non-cavity 57.2 μm long device is ∼ 1.1 Hz, whereas the DCR for the microcavity device is ∼ 0.1 Hz. This confirms another advantage of the microcavity design, in substantially reducing the DCR. Note that a microcavity SNSPD at ∼ 0.9 I C (see vertical dashed line connecting Fig. 3c and Fig. 3d ) maintains its high QE (1.02±8%) over a bias current range for which the DCR stays negligibly small ( ∼ 0.1 Hz); this represents an almost ideal detector performance. The BCR versus bias current curves show QE-like shapes which further suggests it originates from black-body or stray photons rather than being intrinsic to the detectors, like the DCR. This is in agreement with other studies that show how the BCR can be diminished by using well-shielded fibre-coupled cryostats and utilizing inline cold filters [45] , [55] . 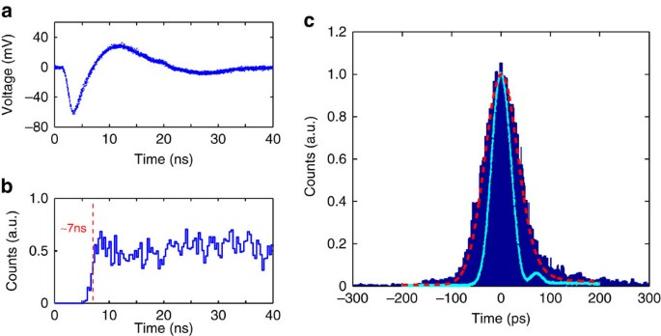Figure 4: Performance of microcavity SNSPDs in time. (a) A single detection pulse measured by a fast oscilloscope. (b) Time histogram of detection events conditioned to a detection event att=0 for a detector excited with a continuous-wave (CW) laser. (c) Time histogram of the detection events for a detector excited with a weak laser pulse (solid cyan line). The red dashed line is the convolution of the laser pulse and the expected instrument response function of the detector. All the measurements of this figure were done for a microcavity detector biased at 3.5 μA. Timing performance characterization Figure 4a shows the electric pulse response of a microcavity SNSPD biased at I B =3.5 μA and excited by a continuous-wave laser. The root-mean-square of the electrical noise is σ n =1.4mV, and the slope of the falling edge is K =51 mV ns −1 . The pulse has a negative polarity to make it compatible with the counter, and shows an under-damped shape because of the frequency cut-offs of the chain of amplifiers (10 MHz to 1.2 GHz). The shape of the response pulse in this readout configuration can be significantly different from the temporal shape of the nanowire bias current, and therefore this setup does not allow a direct estimation of the reset time from the shape of the electrical response (as is traditionally used for estimating the speed of SNSPDs). Instead, the detector reset time is determined by measuring a time histogram of photon detection events conditioned to a detection event at t =0. As shown in Fig. 4b , the detection is restored in ∼ 7 ns after an initial detection event. Figure 4: Performance of microcavity SNSPDs in time. ( a ) A single detection pulse measured by a fast oscilloscope. ( b ) Time histogram of detection events conditioned to a detection event at t =0 for a detector excited with a continuous-wave (CW) laser. ( c ) Time histogram of the detection events for a detector excited with a weak laser pulse (solid cyan line). The red dashed line is the convolution of the laser pulse and the expected instrument response function of the detector. All the measurements of this figure were done for a microcavity detector biased at 3.5 μA. Full size image A schematic of the cryogenic electronic circuit can be seen in Fig. 1 . An inductor, L =100 nH, is externally placed in series with the nanowire and the two are looking at an impedance of R =100 Ω. This roughly makes an electric time-constant of L / R ∼ 1 ns. A reset time on the order of 5 L / R ∼ 5 ns, compatible with the measured value, should therefore be expected. Note a small I B keeps QE ( I B ) away from saturation ( Fig. 3c ), and therefore an easy comparison of the detector reset time and the electrical time constant is possible [60] . The external inductor was used in the measurement set-up to (i) avoid after pulses by allowing a smooth over-damped return of the bias current to the nanowire [61] , and (ii) ensure the stability and low noise performance of the microwave amplifier (LNA in Fig. 1 ) by keeping the impedance seen at its input port closer to the standard value of 50 Ω. However, this inductor can in principle be replaced with a more sophisticated readout circuit to further reduce the reset time to its intrinsic limit, which is known to scale with the nanowire length [47] , [48] , [62] . One estimation of the electronic timing jitter in this setup at I B =3.5 μA is, from Fig. 4a , 2.355 σ n / K =65 ps FWHM. The total timing jitter was directly measured by inserting a microwave intensity modulator (APE of JDSU Inc.) fed by a picosecond pulse generator (Model 4016 of Picosecond Pulse Labs) between the tunable laser and the polarizer of Fig. 1 . The resulting pulsed laser can source fast optical pulses at the peak detection wavelength of any microcavity detector on the chip. A wideband optical/electrical oscilloscope (DCA86100A of Agilent Technologies with Hewlett Packard 83485a plug-in module) synchronized to the electronic trigger output of the pulse generator was used to measure the profile of the optical pulse. The result is a 46 ps FWHM optical pulse (see solid cyan line in Fig. 4c ) with a timing jitter better than a few picoseconds. With these optical pulses applied to a microcavity SNSPD, a total timing jitter measurement obtained using the same oscilloscope resulted in the blue histogram shown in Fig. 4c , with a ∼ 90 ps FWHM. Subtracting the additional jitter due to the finite width of the optical pulses from the measured total jitter yields FWHM as the measured jitter of the detector at I B =3.5 μA. This is close to the above 65 ps estimation of the electronic noise jitter. Convolving the profile of the optical pulse with a 65 ps FWHM Gaussian distribution results in the dashed red line of Fig. 4c which well describes the overall shape of the measured total jitter. Increasing the I B from 3.5 μA to 5.0 μA increased the slope of the falling edge to K =63mV ns −1 , and reduced the total measured jitter to ∼ 72 ps FWHM. This gives a detector jitter of FWHM at I B =5.0 μA which is again close to the value of the electronic timing jitter of 2.355 σ n / K =53 ps FWHM. All these experiments and observations suggest a read-out noise limited performance of the timing jitter for the microcavity SNSPDs, consistent with reports on conventional SNSPDs with comparable bias currents [60] . The energy stored in a microcavity cavity decays with a time constant τ e = Q / ω R . This gives τ e =0.23ps for the microcavity SNSPD designs reported here. Provided τ e is much smaller than the minimum reported timing jitter for nanowire detectors (> ∼ 15 ps), this cavity decay time constant should not have any adverse effect on the timing jitter of microcavity SNSPDs. The demonstrated impact of cavity-based near-perfect absorption on the performance of a single-photon detector paves the way for integrating hundreds of ultrahigh performance detectors on a chip. The silicon host material facilitates high-performance microcavity SNSPDs because of its high index contrast, while also offering the potential of integrating on-chip electronic circuits with the detectors to further boost the performance, and to handle the complexity of scaling up the read-out circuits. This latter point is especially interesting in light of studies that show the compatibility of CMOS transistors with the cryogenic environment [63] , [64] . The speed performance of microcavity SNSPDs combined with their built-in filtered QE, and advanced fibre to waveguide-coupling methods [65] , will also make these detectors ideal for implementing fast quantum communication systems. Simulations Frequency domain finite element solvers (COMSOL, Inc.) are used for numerical simulations. The index of refraction for silicon is set to 3.45 (measured close to 1,550 nm at cryogenic temperatures [66] ), and the environment is assumed to be superfluid helium ( n =1.03). The index of refraction for NbTiN is set to 4.17+i5.62 (ref. 67 ). Eigenmode analysis is used for all Q factor simulations, while the simulated spectra are obtained by using available numeric port boundary conditions. Fabrication The devices were fabricated on NbTiN-coated (8 nm thick—STAR Cryoelectronics Inc.) SOI wafers with a silicon device layer thickness of 200 nm and a buried oxide thickness of 1,220 nm. The superconducting thin film has a critical temperature T C =7.16 K, and critical current density J C ( T =0)=7.57 × 10 6 A cm −2 (see Supplementary Note 3 and Supplementary Fig. 2 for details). Positive electron-beam (e-beam) resist (ZEP520A from ZEON Corp.) was spin-coated at 1,800 r.p.m. and hot-plate backed at 180 °C for 3 min to make a 600 nm thick film. Contact pads and the first set of alignments marks were defined in a 25 KeV e-beam lithography machine (dose 110 μC cm −2 ) and developed in o-xylene at 20 °C for 60 s followed by a 30 s soak in isopropyl alcohol (IPA) and a deionized water rinse. The chip was rinsed in 140:1 BHF:H 2 O for 60 s to wet-etch ∼ 1 nm of NbTiN surface oxides, and was immediately transferred to an e-beam evaporator chamber to deposit an 8 nm/90 nm titanium-gold bilayer, followed by lift-off in sonicated chlorobenzene. The chip was coated again by 600 nm thick ZEP520A, after which the photonic structures and a second set of alignments marks were e-beam written using the original gold alignment marks at 140 μC cm −2 . The sample was then developed in cold o-xylene (4 °C—to improve contrast [68] ). Reactive ion etching (RIE) in 15:2 CF 4 :O 2 30 s and 15:1 CF 4 :O 2 ∼ 300 s was used to vertically etch through the entire thickness of unprotected NbTiN and silicon to yield the NbTiN-coated photonic structures. Spin-coating of 1:1 Anosole:ZEP520A at 2,800 r.p.m. and the same baking conditions were used to coat 180 nm of resist on flat areas and 110 nm on waveguides that are surrounded by relatively deep trenches. The second set of alignment marks were uncovered by e-beam lithography and development to allow sharp imaging of the marks for the last lithography step. The nanowires were written using these uncovered marks at 78 mC cm −2 for which ZEP520A acts as a negative resist [69] . All of the resist except the area exposed by the high-dose e-beam was removed by 5 min exposure to ultraviolet radiation ( λ =320 nm, ∼ 3 W cm −2 ) and a 1 min rinse in chlorobenzene. A final RIE in 15:2 CF 4 :O 2 for ∼ 40 s was used to etch the unprotected NbTiN and 10 nm of silicon. SEM images of several samples indicates this process yields better than ±20 nm alignment of the nanowires with the nanobeam cavities. Four of the reported results in Fig. 3 were obtained from a larger set of 10 devices on a chip, six of which did not work because the measured I C was too small. Measuring η C It is relatively difficult to directly measure η C —the coupling efficiency between the photons incident on the cryostat windows at room temperature and the strip waveguide—as there is no direct means of accessing the strip waveguide inside the cryostat. The Supplementary Information (referenced below) provides a detailed explanation of how η C was laboriously determined by quantifying losses associated with all of the elements between the laser source and the detectors. Another relatively simple method for accurately determining η C is described here. It makes use of several reference structures to calibrate the microcavity devices to within a scaling constant. The first set of test devices are laid out as two grating couplers connected with a long waveguide ( Fig. 1c ) that has a U-shaped nanowire on top (the same nanowire geometry as the TW SNSPD devices presented, but without contacts). Seven of these devices with nanowire lengths ( L NW ) from 0 to 60 μm were made and their transmission ( T ) measured (see Supplementary Note 4 and Supplementary Fig. 3 for full details). A linear fit to log( T / T ( L NW =0)) versus L NW yields η A versus L NW for devices without cavities. At L NW =57.2 μm the measured η A =0.928, and the best linear fit gives 0.917, both in good agreement with the designed η A of 0.90. The results also indicate that the η A is almost wavelength independent within the relatively narrow spectrum of interest. Next, the QE η C =(PCR−BCR)/ R Ph at 1,550 nm for the 57.2-μm long TW SNSPD versus bias current is measured (scaled version of diamonds in Fig. 3c ). Using the best sigmoidal fit to the measured points, the maximum saturated QE η C and QE η C at 0.9 I C were determined and divided to yield , where is the saturated η D of the 57.2 μm device at 1,550 nm. Measuring QE η C versus wavelength at 0.9 I C , equating it to η A η D ( λ ,0.9 I C ) η C =0.917 η D ( λ ,0.9 I C ) η C , and multiplying both sides by the constant η D sat / η D (1,550 nm,0.9 I C )=0.89 −1 , yields . Given the very small range of wavelengths relevant to the data of Fig. 3 , and the results of other studies on SNSPDs that use ultranarrow nanowires [59] , η D ( λ , 0.9 I C )/ η D (1,550 nm, 0.9 I C ) ≃ 1 is expected. Therefore, the present analysis yields which accurately describes the total profile of η C ( λ ) within the scaling constant, . The nice feature of the above procedure is that it almost completely describes η C ( λ ) without need for detailed analysis of the elements that contribute to η C ( λ ) (for example losses of cryostat windows, grating couplers, waveguides and so on). However, the value of , which is essential in determining of the absolute value of on-chip QEs, cannot be directly measured using this calibration method. For this reason, a detailed approach that gives η C ( λ ) and its uncertainty by determining the efficiency of each contributing element is reported in the Supplementary Note 5 and Supplementary Figs 4–11 . The final result in Supplementary Fig. 11 shows η C ( λ ) (red and dashed lines). As can be seen, the detailed approach gives η C with ±8% of uncertainty (corresponding to one s.d.) relative to the mean value for wavelengths close to 1,550 nm. This uncertainty is dominantly determined by the sample to sample variation of the efficiency of the grating couplers ( Supplementary Fig. 8 ). The independently determined as described above is also shown in Supplementary Fig. 11 (blue dots). Note that follows the same spectral shape as η C ( λ ). This validates the assumption that η D ( λ ,0.9 I C ) is independent of wavelength over the small range of relevant wavelengths. That is η D ( λ , 0.9 I C )/ η D (1,550 nm, 0.9 I C ) ≃ 1, as otherwise, would have had a different spectral shape. Also note that almost perfectly overlaps the nominal result for the measured η C , especially for wavelengths close to 1,545 nm (that is, the important wavelength of the peak QE for microcavity SNSPDs in which η C is determined with its minimum variation of ±8%). This coincidence of the directly measured η C , and the obtained using the calibration technique described above, implies that ( to one s.d. of uncertainty). The close to unity is in agreement with other studies on SNSPDs that exhibit a saturated QE( I B ) response [60] , [70] . Finally, the above results provide two essentially identical sets of data that could be used for normalizing the QE η C to QE: one is the mean η C ( λ )±8%, and the other is with . As the data for is less noisy (smoother and less Fabry–Perot like shapes) than that associated with the other more involved determination of η C (compare the two on Supplementary Fig. 11 ), the later set (shown by blue circles in Fig. 3a ) is used as the mean η C throughout the paper. The consistency of measurement and simulation results (for example, high-quality fit of the resonant response to a single Lorentzian line shape in Fig. 3b , the almost flat response of the TW SNSPD in the same figure, and the saturated levels of Fig. 3c at levels expected from simulations) further confirms the validity of this η C . Measuring count rates The count rates (CR) are by definition the number of counts registered by a counter per unit time during which the detector and all the readout electronics are active. Because the counter used in the set-up (PicoHarp 300, PicoQuant Inc.), has a dead time ( T DT ) of 87 ns, in all of the CR measurements reported here, the effect of T DT was included by defining CR=CR m /(1−CR m T DT ), where CR m is simply the number of counts divided by counting time. The linearity of CR with R Ph confirms that the measured CRs are neither affected by T DT or by detector nonlinearities. How to cite this article : Akhlaghi, M. K. et al . Waveguide integrated superconducting single-photon detectors implemented as near-perfect absorbers of coherent radiation. Nat. Commun. 6:8233 doi: 10.1038/ncomms9233 (2015).